Switching of macroscopic molecular recognition selectivity using a mixed solvent system The formation of macroscopic assemblies based on molecular recognition is promising in a wide variety of fields of materials science. Switching of the selectivity of macroscopic assemblies is of increasing importance to produce highly functional materials. Here we show macroscopic assembly based on molecular recognition using polyacrylamide gel modified with pyrenyl (Py) moiety (Py-gel) and gels possessing CD moieties (αCD-gel, βCD-gel and γCD-gel) in a mixed solvent of water and dimethyl sulfoxide. Changing the composition of the mixed solvent can switch the selectivity of Py-gel, because the fractions of the monomer and dimer of the Py moieties on the gel surface depend on the mixed solvent composition. The monomer and dimer of the Py moieties prefer βCD and γCD moieties, respectively. On the basis of microscopic molecular recognition of a number of biological molecules, living organisms are ubiquitous macroscopic assemblies formed from supramolecular structures [1] , [2] , [3] . In various materials science fields, macroscopic assemblies in artificial systems based on microscopic molecular recognition are promising, for example, self-healing materials [4] , [5] , [6] . However, construction of artificial macroscopic assemblies based on molecular recognition remains a great challenge. Previously, we have reported macroscopic molecular recognition using a simple system of a polyacrylamide-based hydrogel possessing cyclodextrin (CD) and guest moieties [7] , [8] , [9] . According to their binding affinities, gels possessing αCD, βCD and γCD moieties recognize gels possessing their respective counterparts. Recently, we have focussed on macroscopic observations of molecular recognition using aromatic compounds because aromatic compounds absorb light and consequently, may transfer energy and electrons. We have reported that a gel possessing βCD moieties can discriminate the substitution position on a naphthyl group with the appropriate contents of βCD and naphthyl moieties, although these moieties have similar binding constants [10] . More recently, we have reported selective photoresponsive switching of macromolecular recognition using an azobenzene moiety [11] . Pyrene is a popular fluorophore because it emits fluorescence with a relatively high quantum yield in both its monomer and dimer states [12] . On the other hand, pyrene is highly hydrophobic; its solubility in water is very low (<10 −6 M) and easily forms dimers and aggregates in aqueous media [13] , [14] . In the present study, we modified a polyacrylamide gel with pyrenyl (Py) moiety (Py-gel) and investigated its interaction with gels possessing CD moieties (αCD-gel, βCD-gel and γCD-gel) ( Fig. 1 ), using a mixed solvent of water and dimethyl sulfoxide (DMSO). The selectivity of Py-gel can be switched by varying the volume fraction of DMSO in the mixed solvent system ( x DMSO ). 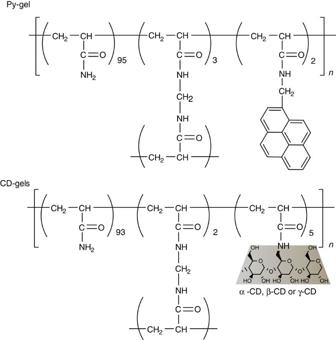Figure 1: Chemical structures of Py-gel and CD-gels. CD-gels were αCD-gel, βCD-gel and γCD-gel. Mol% are those in monomer feed, which are nearly identical to those in the obtained polymer gel. Figure 1: Chemical structures of Py-gel and CD-gels. CD-gels were αCD-gel, βCD-gel and γCD-gel. Mol% are those in monomer feed, which are nearly identical to those in the obtained polymer gel. Full size image Preparation of Py-gel and CD-gels The gels used in the present study were prepared by conventional radical terpolymerization of acrylamide, N , N ′-methylenebis(acrylamide) and a monomer possessing a Py or CD moiety ( Fig. 1 ). During gel preparation, water was used as the solvent for CD-gels, while DMSO was used as the solvent for the Py-gel owing to the solubility of the Py monomer in water. After gel preparation, DMSO was replaced with water for the Py-gel. Interaction of Py-gel with CD-gels in the mixed solvent. The interaction of Py-gel with CD-gels was investigated by shaking gel pieces in a mixed solvent of water and DMSO with various volume fractions of DMSO ( x DMSO ), as can be seen in Fig. 2 . At x DMSO =0, Py-gel pieces interact only with γCD-gel pieces to form a gel assembly ( Fig. 2a ), and the resulted gel assembly is sufficiently stable to be picked up ( Supplementary Fig. S1 ). At x DMSO =0.2, Py-gel pieces interact with both βCD-gel and γCD-gel pieces to form a larger assembly ( Fig. 2b ). As x DMSO increases up to 0.5, Py-gel pieces interact with βCD-gel pieces, but not the γCD-gel pieces ( Fig. 2c ). At x DMSO =1, Py-gel pieces and CD-gel pieces do not interact. Furthermore, Py-gel pieces do not interact with αCD-gel pieces regardless of x DMSO because αCD is too small to include the Py moiety. These observations indicate the selectivity of Py-gel strongly depends on the composition of the mixed solvent system. Py-gel prefers γCD-gel at x DMSO =0. Py-gel interacts with both βCD-gel and γCD-gel at x DMSO =0.2. However, Py-gel prefers βCD-gel at x DMSO =0.5. Thus, adjusting the mixed solvent composition can switch the selectivity of Py-gel, allowing macroscopic discrimination of αCD-, βCD- and γCD-gel. 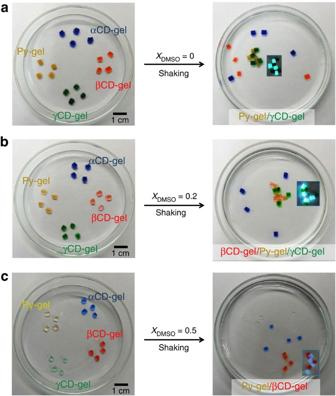Figure 2: Pictures of the interaction of Py-gel (yellow) with αCD-gel (blue), βCD-gel (red) and γCD-gel (green) in a glass petri dish. (a) Py-gel pieces interact with γCD-gel pieces atxDMSO=0. (b) Py-gel pieces assemble with both βCD-gel and γCD-gel pieces atxDMSO=0.2. (c) Py-gel pieces prefer βCD-gel pieces atxDMSO=0.5. The insets were taken under irradiation with 365 nm light. The interaction between Py-gel and αCD-gel was not observed. Scale bar, 1.0 cm. Figure 2: Pictures of the interaction of Py-gel (yellow) with αCD-gel (blue), βCD-gel (red) and γCD-gel (green) in a glass petri dish. ( a ) Py-gel pieces interact with γCD-gel pieces at x DMSO =0. ( b ) Py-gel pieces assemble with both βCD-gel and γCD-gel pieces at x DMSO =0.2. ( c ) Py-gel pieces prefer βCD-gel pieces at x DMSO =0.5. The insets were taken under irradiation with 365 nm light. The interaction between Py-gel and αCD-gel was not observed. Scale bar, 1.0 cm. Full size image The interaction strength of the gels was investigated by stress−strain measurements using a tensile meter. A gel assembly of Py-gel and CD-gel cubes was set on a tensile meter, and the stress was monitored as a strain was applied ( Supplementary Fig. S2 ). Using the stress−strain data, Fig. 3 plots the stress at rupture as a function of x DMSO . For Py-gel/γCD-gel assemblies, the stress at rupture decreases as x DMSO increases with a shoulder at x DMSO ~0.4. In contrast, the stress at rupture increases for Py-gel/βCD-gel assemblies as x DMSO increases, reaches a maximum at x DMSO ~ 0.4, and then decreases. These observations confirm selectivity of Py-gel switches; Py-gel prefers γCD-gel at x DMSO <0.2. At x DMSO ~0.2, Py-gel interacts with both βCD-gel and γCD-gel. At 0.2 < x DMSO ≤0.6, Py-gel prefers βCD-gel. However, at x DMSO =1, Py-gel does not interact with CD-gels because inclusion complexes are not formed in DMSO. 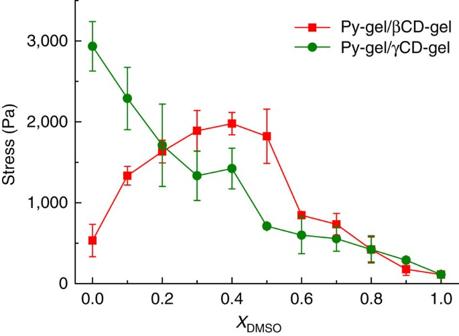Figure 3: Stress at rupture as a function ofxDMSOfor the Py-gel/βCD-gel (red) and Py-gel/γCD-gel assemblies (green). Py-gel prefers γCD-gel atxDMSO<0.2. AtxDMSO~0.2, Py-gel interacts with both βCD-gel and γCD-gel. At 0.2 <xDMSO≤0.6, Py-gel prefers βCD-gel. AtxDMSO=1, Py-gel does not interact with CD-gels. Stress-strain measurements were repeated at least three times, and the error bars denote the standard deviations. Figure 3: Stress at rupture as a function of x DMSO for the Py-gel/βCD-gel (red) and Py-gel/γCD-gel assemblies (green). Py-gel prefers γCD-gel at x DMSO <0.2. At x DMSO ~0.2, Py-gel interacts with both βCD-gel and γCD-gel. At 0.2 < x DMSO ≤0.6, Py-gel prefers βCD-gel. At x DMSO =1, Py-gel does not interact with CD-gels. Stress-strain measurements were repeated at least three times, and the error bars denote the standard deviations. Full size image Fluorescent study on the model systems To understand the selectivity switching mechanism, fluorescence measurements were carried out using a model polymer, that is, polyacrylamide modified with a 1-mol% Py moiety (pAAm/Py, Supplementary Fig. S3 ). Supplementary Fig. S4a shows the steady-state fluorescence spectra of pAAm/Py at various x DMSO in the absence of CD. At x DMSO =0, the spectrum exhibits monomer fluorescence in the region of 360–380 nm and an excimer emission around 485 nm. The Py content of pAAm/Py is relatively low, but Py moieties easily form dimers within the same polymer chain owing to hydrophobicity. As x DMSO increases, the intensity of the excimer emission decreases until almost disappears at x DMSO >0.8. The ratio ( I E / I M ) of the fluorescence intensities around 376 and 485 nm, which are ascribed predominantly to monomer and excimer emissions, respectively, were calculated and plotted against x DMSO ( Supplementary Fig. S4b ). I E / I M decreases as x DMSO increases and reaches ca. 0.02 at x DMSO >0.8. The same x DMSO dependency of I E / I M occurs in the fluorescence spectra of Py-gel ( Supplementary Fig. S5 ), indicating that the addition of DMSO makes the Py moiety more solvophilic and inhibits the formation of the excimer. In addition, insets in Fig. 2 visibly indicate the formation of the dimer in Py-gel at x DMSO =0 (bluish green light emission) and the monomer at x DMSO =0.5 (blue light emission) under photoirradiation. Fluorescence spectra were also measured for pAAm/Py at x DMSO =0, 0.2, 0.5 and 1 in the presence of various concentrations of βCD or γCD to understand the effects of x DMSO on the interaction of the Py moiety with βCD or γCD ( Supplementary Fig. S6 ). At x DMSO =0, the fluorescence spectra for pAAm/Py are nearly independent of the βCD concentration. On the other hand, as γCD concentration increases, the intensity of the monomer fluorescence decreases while the intensity of excimer emission increases, demonstrating that the Py moiety interacts with γCD in its dimer state but not βCD at x DMSO =0. At x DMSO =0.2, the intensity of the monomer fluorescence increases as βCD increases. On the other hand, the intensity of the excimer fluorescence slightly increases as γCD increases. These observations indicate that the Py moiety interacts with βCD in its monomer state, but with γCD in its dimer state at x DMSO =0.2. At x DMSO =0.5, the intensity of monomer fluorescence increases as βCD increases, but the fluorescence spectra are almost independent of the γCD concentration, indicating that the Py moiety interacts only with βCD. In addition, at x DMSO =1, that is, in DMSO, the spectra do not change on the further addition of βCD or γCD. Consistent with previous findings [15] , [16] , these observations lead to the conclusion that the Py moiety interacts with βCD in its monomer state to form a 1:1 complex, whereas the Py moiety interacts with γCD in its dimer state to form a 2:1 complex. On the basis of the characterization data, the selectivity switching mechanism for the Py-gel dependence on x DMSO is considered ( Fig. 4 ). At x DMSO =0, a significant fraction of the Py moieties on the Py-gel surface form dimers and interact with γCD moieties on the γCD-gel. In contrast, at x DMSO =0, the fraction of the monomer Py moiety on the Py-gel surface is too low to interact with the βCD moieties on the βCD-gel surface. At x DMSO =0.2, the Py moiety is slightly solvophilic, and the fractions of monomer and dimer of the Py moieties on the gel surface are sufficient to interact with both βCD-gel and γCD-gel to form larger assemblies containing all three types of pieces. At x DMSO =0.5, the formation of dimer Py moieties on the Py-gel surface is insignificant, but the monomer Py moieties still interact with βCD moieties on the βCD-gel surface. Thus, Py-gel interacts only with the βCD-gel. 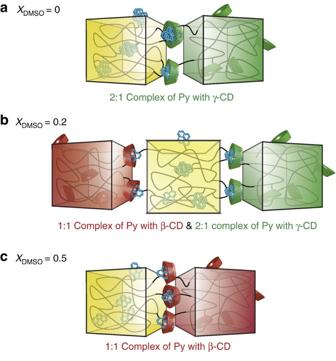Figure 4: Conceptual illustrations for selectivity switching of Py-gel as a function ofxDMSO. (a) AtxDMSO=0, Py dimers are formed and included by γCD on the interface. (b) AtxDMSO=0.2, Py monomers and dimers coexist in the gel that interact with both βCD and γCD. (c) AtxDMSO=0.5, Py dimers are separated into monomers that included by βCD on the interface of gel assembly. Gels in yellow, red and green colour represent Py-gel, βCD-gel and γCD-gel, respectively. Figure 4: Conceptual illustrations for selectivity switching of Py-gel as a function of x DMSO . ( a ) At x DMSO =0, Py dimers are formed and included by γCD on the interface. ( b ) At x DMSO =0.2, Py monomers and dimers coexist in the gel that interact with both βCD and γCD. ( c ) At x DMSO =0.5, Py dimers are separated into monomers that included by βCD on the interface of gel assembly. Gels in yellow, red and green colour represent Py-gel, βCD-gel and γCD-gel, respectively. Full size image In conclusion, the selectivity of Py-gel can be switched by changing the composition of the mixed solvent system composed of water and DMSO, because the monomer and dimer fractions of the Py moieties on the gel surface depend on x DMSO ; the monomer and dimer of Py moieties prefer the βCD and γCD moieties, respectively. These observations allow the macroscopic discrimination of αCD-gel, βCD-gel and γCD-gel using Py-gel. Measurements 1 H NMR spectra were measured on a JEOL JNM-ECA500 spectrometer, and chemical shifts were referenced to the solvent values (2.49 and 4.79 p.p.m. for DMSO- d 6 and D 2 O, respectively). Positive-ion matrix-assisted laser desorption/ionization time-of-flight mass spectrometry experiments were performed using a Shimadzu/KRATOS Axima CFR Ver.2.2.3 mass spectrometer calibrated by α-cyano-4-hydroxycinnamic acid and insulin. Fluorescence spectra were obtained on a HITACHI F-2500 spectrophotometer, using a 1-cm quartz cuvette. The slit widths for both excitation and emission sides were kept at 2.5 nm during measurement. All fluorescence spectra were reported as averages of three scans with an error less than 5%. The stress-strain curves for gel assemblies were recorded using a Yamaden RE-33005 Rheoner creep meter. Each sample (5×10 mm 2 in size) was measured at a rate of 0.1 mm s −1 at room temperature. Materials 1-Pyrenemethylamine hydrochloride was purchased from Sigma-Aldrich. Acryloyl chloride was obtained from Tokyo Chemical Industry. Triethylamine, acrylamide (AAm), ammonium peroxodisulfate (APS), N , N , N ′, N ′-tetramethylethylenediamine (TMEDA), N , N ′-methylenebis(acrylamide) (MBA), acetone, methanol, DMSO (spectra grade), NaHCO 3 and NaOH were purchased from Nacalai Tesque. N , N -Dimethylformamide and dichloromethane (DCM) were purified by utilizing a Glass Contour solvent dispensing system. Water was purified by a Millipore Milli-Q system. Cyclodextrins (αCD, βCD and γCD) were purchased from Junsei Chemical. and recrystallized twice from water before using. Mono(6-deoxyacrylamido)-α-cyclodextrin (A6αCD), mono(6-deoxyacrylamido)-β-cyclodextrin (A6βCD) and mono(6-deoxyacrylamido)-γ-cyclodextrin (A6γCD) were prepared according to the procedure reported previously [10] , [17] . Other reagents were reagent grade and used without further purification. Preparation of N -(1-pyrenylmethyl)acrylamide (A1Py) To a solution of 1-pyrenemethylamine hydrochloride (1.07 g, 4.00 mmol) and acryloyl chloride (0.95 ml, 12 mmol) in DCM (55 ml), a solution of triethylamine (1.62 ml, 16.0 mmol) in DCM (5.0 ml) solution was added dropwise at 0 °C. The reaction was allowed to run overnight at room temperature. After evaporation of the solvent, A1Py was purified by silica gel column chromatography using a mixed solvent of ethyl acetate and hexane (1/3, v/v) and obtained as a pale yellow powder: yield 390 mg, 34 %; mp 215–216 °C; 1 H NMR (500 MHz, DMSO- d 6 , 30 °C) δ 8.759 (brs, 1H, NH), 8.382 (d, J =9.2 Hz, 1H, pyrene), 8.320–8.231 (m, 4H, pyrene), 8.156 (s, 2H, pyrene), 8.073 (t, J =7.6 Hz, 1H, pyrene), 8.038 (d, J =7.7 Hz, 1H, pyrene), 6.312 (dd, J =17.1 and 10.1 Hz, 1H, vinyl), 6.185 (dd, J =17.1 and 2.3 Hz, 1H, vinyl), 5.630 (dd, J =10.1 and 2.4 Hz, 1H, vinyl), 5.093 (d, J =5.8 Hz, 2H, CH 2 ). 13 C NMR (125 MHz, DMSO- d 6 , 30 °C) δ 164.44 (C=O), 132.58 (PyC 1 ), 131.56 (PyC 11 ), 130.74 (C=C), 130.26 (PyC 14 ), 130.17 (C=C), 128.16 (PyC 10 ), 127.59 (PyC 13 ), 127.31 (PyC 12 ), 127.04 (PyC 6 ), 126.88 (PyC 5 ), 126.21 (PyC 9 ), 125.54 (PyC 8 ), 125.23 (PyC 3 ), 125.14 (PyC 7 ), 124.69 (PyC 2 ), 124.04 (PyC 16 ), 123.88 (PyC 15 ), 123.15 (PyC 4 ), 40.46 (C-N). Anal. Calcd for C 20 H 15 NO(H 2 O) 0.13 : C, 83.50; H, 5.35; N, 4.87. Found: C, 83.50; H, 5.34; N 4.89. Positive ion matrix-assisted laser desorption/ionization time-of-flight mass spectrometry: m / z =285.1, [M+H + ] 285.2. Preparation of a model polymer (pAAm/Py) A predetermined amount of AAm and A1Py were dissolved in dimethylformamide. After purging with dry argon for 30 min, APS (3 mg, 1×10 −5 mol) was added to the monomer solution. The reaction mixture was placed into a cuvette equipped with a stirrer and sealed. The cuvette was warmed with an oil bath thermostated at 60 °C overnight. The reaction mixture was poured into excess of methanol to give a precipitate. The polymer obtained was recovered by filtration and dried under vacuum. Preparation of Py-gel A predetermined amount of AAm (405.2 mg, 5.70 mmol), MBA (27.8 mg, 0.18 mmol) and A1Py (34.2 mg, 0.12 mmol) were dissolved in DMSO (3.0 ml). After purging with dry argon for 30 min, APS (6 mg, 3×10 −5 mol) was added to the monomer solution. The reaction mixture was placed into a 1-cm quartz cuvette and sealed. The cuvette was set into a 60-°C oven for 8 h. The gel was washed with DMSO and soaked in excess of the solvent used. Preparation of CD-gels A predetermined amount of AAm, MBA and a CD monomer (A6αCD, A6βCD or A6γCD) were dissolved in water (2.0 ml) in a 1-cm quartz cuvette. After addition of APS (3 mg, 1×10 −5 mol) and TMEDA (2.5 μl, 2×10 −5 mol), the reaction mixture immediately turned into a gel, which was washed with water to remove unreacted monomers and initiators. αCD-gel, βCD-gel and γCD-gel were dyed with blue (Coomassie brilliant blue R-250), red (food pigment red NO.102) and green (cyan NO.1 and yellow NO.4) dyes, respectively, by immersing into a solution of the corresponding dye. The CD-gels were then immersed in excess of the solvent used. How to cite this article: Zheng, Y. et al . Switching of macroscopic molecular recognition selectivity using a mixed solvent system. Nat. Commun. 3:831 doi: 10.1038/ncomms1841 (2012).